Acquisition of innate-like microbial reactivity in mucosal tissues during human fetal MAIT-cell development Innate-like, evolutionarily conserved MR1-restricted mucosa-associated invariant T (MAIT) cells represent a large antimicrobial T-cell subset in humans. Here, we investigate the development of these cells in second trimester human fetal tissues. MAIT cells are rare and immature in the fetal thymus, spleen and mesenteric lymph nodes. In contrast, mature IL-18Rα + CD8αα MAIT cells are enriched in the fetal small intestine, liver and lung. Independently of localization, MAIT cells express CD127 and Ki67 in vivo and readily proliferate in response to Escherichia coli in vitro . Maturation is accompanied by the gradual post-thymic acquisition of the PLZF transcription factor and the ability to produce IFNγ and IL-22 in response to bacteria in mucosa. Thus, MAIT cells acquire innate-like antimicrobial responsiveness in mucosa before exposure to environmental microbes and the commensal microflora. Establishment of this arm of immunity before birth may help protect the newborn from a range of pathogenic microbes. Mucosa-associated invariant T (MAIT) cells are a recently described subset of unconventional, innate-like T cells that are highly abundant in mucosal tissues, liver and peripheral blood [1] , [2] , [3] , [4] . In humans, MAIT cells express a semi-invariant T-cell receptor (TCR), including Vα7.2 coupled with Jα33 segment and a restricted Vβ repertoire, and recognize antigens in complex with the MHC-Ib-related protein (MR1) [2] , [4] . MR1 displays an extraordinary level of evolutionary conservation among placental and marsupial mammals [4] , [5] , [6] , strongly supportive of the notion that MR1 and MAIT cells perform critical functions in the immune system. MAIT cells in peripheral blood are defined by the high expression of CD161, the IL-18 receptor α subunit (IL-18Rα), and the transcription factor ZBTB16 (ref. 7 ), also known as promyelocytic leukaemia zinc-finger protein (PLZF) [8] , [9] . The vast majority of MAIT cells are either CD8αα or CD8αβ, with some CD4 + or CD8/4 double-negative populations [8] , [9] , [10] , [11] . MAIT cells recognize microbial vitamin B 2 (riboflavin) metabolites from a wide range of microbes presented by MR1 molecules [12] , [13] . Recognition of MR1 is dependent on the complementarity determining region (CDR) 1α, CDR2α and CDR3α of the TCR Vα7.2 segment [14] . Once activated by antigen, MAIT cells rapidly produce pro-inflammatory cytokines, including IFNγ, TNF and IL-17 (refs 8 , 10 , 11 , 15 ). This mixed TH1/17 profile most probably contributes to the reported role of MAIT cells in the protection against diverse bacterial and mycobacterial infections in animal models, as well as in human pulmonary tuberculosis [8] , [16] , [17] , [18] , [19] . Whereas MAIT cells probably do not directly recognize viral antigens, indirect involvement of these cells in viral immunopathogenesis can occur, as recently described for HIV-1 infection [11] , [15] , [20] . The development of MAIT cells is currently incompletely understood. In mice, MAIT cells are selected by MR1-expressing cells in the thymus and exit as naive cells [9] . MR1 is ubiquitously expressed by different cells and tissues [5] , [21] , but only transiently visit the plasma membrane [22] . In humans, MAIT cell selection in the thymus is probably dependent on MR1-endogenous ligand-expressing thymocytes [23] . The naive murine MAIT-cell population expands and acquires an effector memory-like phenotype in the periphery after birth, and this process appears to be dependent on both commensal gut floras and on B lymphocytes (reviewed in ref. 1 ). Whether similar conditions are required for MAIT-cell development in humans is unknown. However, human MAIT cells obtained from postnatal thymus and umbilical cord blood display a naive phenotype [9] and readily proliferate following TCR engagement [24] . In contrast, peripheral blood MAIT cells from adults have poor proliferative capacity following TCR stimulation in the absence of exogenous cytokines [3] , [10] , [24] , [25] . The development of human MAIT cells before birth and their relationship to the establishment of mucosal microbiota is currently unknown. In this study, we investigate this central aspect of MAIT-cell immunobiology in second trimester human fetal tissues. The findings define the gradual maturation pathway of MAIT cells in lymphoid and peripheral organs. Furthermore, the data demonstrate the acquisition of innate-like antimicrobial activity of MAIT cells in human fetal intestinal mucosa in utero , before the establishment of the commensal microflora and before exposure to, and priming by, environmental microbes. Identification of PLZF lo MAIT cells in human fetal thymus To investigate the developmental immunobiology of MAIT cells, we prepared mononuclear cell (MNC) single-cell suspensions from second trimester human fetal tissues and devised a flow cytometric gating strategy identifying MAIT cells as CD45 hi CD3 + CD161 hi TCR Vα7.2 + cells ( Supplementary Fig. 1a ). Employing this strategy for identification, MAIT cells were found to be present in human fetal thymi, in both CD3 lo and CD3 hi thymocyte fractions, as a predominantly CD8 + single-positive (SP) population ( Fig. 1a ). This was in contrast to Vα7.2 + CD161 − and Vα7.2 − thymocytes that were present as predominantly CD4 + CD8 + double-positive (DP) populations among the CD3 lo thymocytes, and as mixed CD4 + SP, CD8 + SP and CD4 + CD8 + DP populations among the CD3 hi thymocytes ( Fig. 1a ). The fetal thymic MAIT cells did not express appreciable levels of the MAIT-cell maturation-associated transcription factor PLZF ( Fig. 1a ). These data demonstrate that MAIT cells are present in the fetal thymus and suggest that maturation and acquisition of PLZF-dependent effector functions does not occur intrathymically. 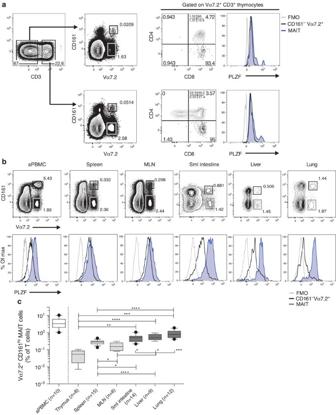Figure 1: Identification and characterization of MAIT cells in second trimester human fetal tissues. (a) Vα7.2+CD161hiMAIT cells identified in CD3loand CD3hithymocytes from eight fetal thymi. The expression of CD4, CD8 and PLZF in these cells was compared with the Vα7.2+CD161−T-cell population (grey rectangular gates). Black dot plots denote Vα7.2+CD161hiMAIT cells and grey contour plots indicate Vα7.2+CD161−T cells. (b) MAIT cells and their PLZF expression in the fetal spleen, mesenteric lymph node (MLN), small (sml) intestine, liver and lung samples, and adult (a) PBMCs as controls. Representative FACS plots are shown. (c) MAIT-cell frequencies in aPBMC (n=10), fetal thymus (n=8), spleen (n=15), MLN (n=8), sml intestine (n=14), liver (n=9) and lung (n=12). Box and whisker plot shows median, IQR and the 10th to the 90th percentile. *P<0.05, **P<0.01, ***P<0.001, ****P<0.0001 (one-way ANOVA followed by Bonferroni’spost hoctest). Figure 1: Identification and characterization of MAIT cells in second trimester human fetal tissues. ( a ) Vα7.2 + CD161 hi MAIT cells identified in CD3 lo and CD3 hi thymocytes from eight fetal thymi. The expression of CD4, CD8 and PLZF in these cells was compared with the Vα7.2 + CD161 − T-cell population (grey rectangular gates). Black dot plots denote Vα7.2 + CD161 hi MAIT cells and grey contour plots indicate Vα7.2 + CD161 − T cells. ( b ) MAIT cells and their PLZF expression in the fetal spleen, mesenteric lymph node (MLN), small (sml) intestine, liver and lung samples, and adult (a) PBMCs as controls. Representative FACS plots are shown. ( c ) MAIT-cell frequencies in aPBMC ( n =10), fetal thymus ( n =8), spleen ( n =15), MLN ( n =8), sml intestine ( n =14), liver ( n =9) and lung ( n =12). Box and whisker plot shows median, IQR and the 10th to the 90th percentile. * P <0.05, ** P <0.01, *** P <0.001, **** P <0.0001 (one-way ANOVA followed by Bonferroni’s post hoc test). Full size image Enrichment of PLZF hi MAIT cells in fetal mucosal tissues We next extended these investigations to the secondary lymphoid organs, the spleen and mesenteric lymph nodes (MLN), as well as the peripheral organs small intestine, the liver and lung. MAIT cells were present in all of these tissues, at varying frequencies ( Fig. 1b,c ). In these fetal tissues, the lung contained the highest percentage of MAIT cells (mean % of CD3 + T cells ±s.d.=0.89±0.48), followed by the liver (0.58±0.23), small intestine (0.54±0.26), spleen (0.28±0.08), MLN (0.17±0.09) and thymus (0.05±0.03) ( Fig. 1c ). Similar to adult peripheral blood MAIT cells, fetal MAIT cells were predominantly CD8 + , alongside with a smaller DN population. Interestingly, the MAIT cell population in the fetal intestine also contained a significant CD4 + subset ( Supplementary Fig. 1b ). There was no significant correlation between gestational age and MAIT cell frequency in the fetal tissues examined. Interestingly, MAIT-cell expression of PLZF at the secondary lymphoid sites spleen and MLN was clearly detectable and higher than in the thymus ( Fig. 1b ). A further enhancement of PLZF expression was evident in the small intestine, liver and lung ( Fig. 1b ). Taken together, these results demonstrate that MAIT cells are present in second trimester fetal tissues with enrichment in mucosal tissues and the liver. This enrichment in peripheral sites occurs concomitantly with a gradual acquisition of PLZF expression during post-thymic maturation. Fetal MAIT cells mature in mucosal tissues and liver Co-expression of high levels of IL-18Rα with the Vα7.2 TCR has been proposed as an alternative way to unequivocally identify MAIT cells [3] , [9] . Indeed, peripheral blood Vα7.2 + CD161 hi MAIT cells obtained from healthy adult individuals almost universally co-expressed IL-18Rα ( Fig. 2a,b and refs 8 , 9 , 11 ). We therefore investigated the expression of IL-18Rα in fetal MAIT cells. Surprisingly, only a small proportion of fetal thymic Vα7.2 + CD161 hi MAIT cells co-expressed IL-18Rα (mean % of Vα7.2 + CD161 hi MAIT±s.d.=39.0±8.7), with similar proportions in the spleen and MLN (48.5±13.9 and 33.9±10.5, respectively) ( Fig. 2a,b ). In contrast, IL-18Rα was co-expressed by most, but not all, Vα7.2 + CD161 hi MAIT cells in the small intestine (87.4±6.1), liver (80.5±16.4) and lung (82.9±12.0) ( Fig. 2a,b ). These results indicate that IL-18Rα + PLZF + MAIT cells are enriched in fetal mucosal tissues and liver. 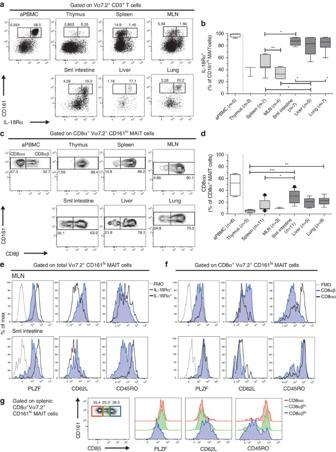Figure 2: Maturation and acquisition of IL-18Rα and CD8αα in fetal mucosal and liver MAIT cells. (a) IL-18Rα and CD161 co-expression was determined on Vα7.2+CD3+T cells from fetal tissues and adult PBMCs. (b) Frequency of IL-18Rα co-expression in fetal Vα7.2+CD161hiMAIT cells from the thymus (n=3), spleen (n=7), MLN (n=4), small (sml) intestine (n=7), liver (n=5) and lung (n=7), in comparison with adult (a) PBMC (n=5). (c,d) Identification and enumeration of the CD8αα MAIT-cell subset within fetal CD8α+Vα7.2+CD161hiMAIT cells in the thymus (n=5), spleen (n=11), MLN (n=3), sml intestine (n=11), liver (n=5) and lung (n=9), in comparison with aPBMC (n=6). (e–g) PLZF, CD62L and CD45RO expression determined in IL-18Rα−and IL-18Rα+Vα7.2+CD161hiMAIT cells, and in CD8αα and CD8αβ MAIT cells from three independent, matched fetal MLN and small intestine samples, and on CD8αα, CD8αβloand CD8αβhiMAIT cells from five independent fetal spleens. Representative FACS plots are shown. Box and whisker plot shows median, IQR and the 10th to the 90th percentile. *P<0.05, **P<0.01, ***P<0.001 (Kruskal–Wallis ANOVA followed by Dunn’spost hoctest). Figure 2: Maturation and acquisition of IL-18Rα and CD8αα in fetal mucosal and liver MAIT cells. ( a ) IL-18Rα and CD161 co-expression was determined on Vα7.2 + CD3 + T cells from fetal tissues and adult PBMCs. ( b ) Frequency of IL-18Rα co-expression in fetal Vα7.2 + CD161 hi MAIT cells from the thymus ( n =3), spleen ( n =7), MLN ( n =4), small (sml) intestine ( n =7), liver ( n =5) and lung ( n =7), in comparison with adult (a) PBMC ( n =5). ( c , d ) Identification and enumeration of the CD8αα MAIT-cell subset within fetal CD8α + Vα7.2 + CD161 hi MAIT cells in the thymus ( n =5), spleen ( n =11), MLN ( n =3), sml intestine ( n =11), liver ( n =5) and lung ( n =9), in comparison with aPBMC ( n =6). ( e – g ) PLZF, CD62L and CD45RO expression determined in IL-18Rα − and IL-18Rα + Vα7.2 + CD161 hi MAIT cells, and in CD8αα and CD8αβ MAIT cells from three independent, matched fetal MLN and small intestine samples, and on CD8αα, CD8αβ lo and CD8αβ hi MAIT cells from five independent fetal spleens. Representative FACS plots are shown. Box and whisker plot shows median, IQR and the 10th to the 90th percentile. * P <0.05, ** P <0.01, *** P <0.001 (Kruskal–Wallis ANOVA followed by Dunn’s post hoc test). Full size image We next examined the frequency of CD8αα MAIT cells in fetal tissues, as recent studies have shown that the CD8αα subset represents a significant proportion of CD8 + (that is, CD8α + ) MAIT cells in healthy adults [10] . While half of adult peripheral blood CD8α + Vα7.2 + CD161 hi MAIT cells were CD8αα (50.0±17.4%), only very small proportions of fetal thymic CD8α + Vα7.2 + CD161 hi MAIT cells were CD8αα (5.3±2.2%), with comparable levels in the spleen and MLN (13.8±9.1% and 10.1±1.1%, respectively) ( Fig. 2c,d ). Interestingly, the proportion of the CD8αα subset within CD8α + Vα7.2 + CD161 hi MAIT cells was significantly higher in the small intestine (28.2±10.8%), liver (19.0±8.3%) and lung (22.1±7.2%). These results indicate that similar to the data on IL-18Rα expression, the CD8αα phenotype is also preferentially enriched in fetal MAIT cells located in mucosal tissues and the liver. Because both IL-18Rα expression and the CD8αα phenotype were concomitantly acquired in fetal mucosal tissues and the liver, we examined whether these markers were linked with fetal MAIT-cell maturation in vivo . Expression of PLZF, CD62L and CD45RO, which is associated with a mature MAIT-cell phenotype in adult PBMC [3] , [9] , [10] , was determined in three matched MLN and small intestine tissue samples. In the MLN, IL-18Rα + Vα7.2 + CD161 hi MAIT cells expressed higher levels of PLZF and CD45RO, but lower levels of CD62L, than those of IL-18Rα − Vα7.2 + CD161 hi MAIT cells ( Fig. 2e ). A similar pattern was noted in the small intestine, with even higher PLZF and CD45RO levels in the IL-18Rα + population ( Fig. 2e ). Similarly, CD8αα MAIT cells in the MLN also displayed higher PLZF and CD45RO levels, and lower CD62L expression, as compared with the CD8αβ MAIT cells, although these patterns were less obvious in the small intestine ( Fig. 2f ). We then investigated further the expression of these maturation markers in all CD8α + MAIT subsets (CD8αα, CD8αβ lo , CD8αβ hi ) in fetal spleen where the abundance of MNCs allowed us to perform detailed ex vivo analyses that were not possible in other organs. CD8αβ lo MAIT cells had already started acquiring a mature PLZF hi , CD62 int , CD45RO hi phenotype ( Fig. 2g ). These results suggest that fetal CD8αα MAIT cells may be derived from CD8αβ MAIT cells in a stepwise CD8αβ hi → CD8αβ lo → CD8αα (CD8αβ − ) manner. These observations are consistent with other studies suggesting that CD8αα T cells are derived from the CD8αβ T-cell population extra-thymically [10] , [26] . Taken together, our results suggest that fetal IL-18Rα + and CD8αα MAIT cells are more mature than their IL-18Rα − and CD8αβ counterparts, respectively, and that this relatively mature fetal MAIT subset is preferentially located in fetal mucosal tissues and liver. Activated memory-like MAIT cells in the small intestine We next characterized fetal tissue MAIT cells in more detail with regard to activation and maturation markers. MAIT cells from fetal thymi, spleens and MLNs did not express appreciable levels of the activation marker CD25, whereas CD25 was clearly detectable on MAIT cells in small intestine, and to some extent in the liver and lung ( Fig. 3a ). CD45RO was expressed at low levels in the thymus, spleen and MLN, but at higher levels in the small intestine, liver and lung ( Fig. 3a,b ), irrespective of IL-18Rα or CD8α co-expression ( Fig. 2 ). The opposite pattern was observed for CD62L and to some extent also for CCR7, with higher levels in the thymus, spleen and MLN, and lower expression in the small intestine, liver and lung ( Fig. 3a,b ). CD127 (IL-7Rα) was consistently expressed by MAIT cells derived from different fetal tissues ( Fig. 3a ), an observation in line with a role for IL-7 in MAIT-cell development, in addition to its recently described role in regulating the function of MAIT cells in adult peripheral blood [27] . CCR9, which is involved in recruitment to the gastrointestinal tract, was expressed by some thymic MAIT cells and the majority of small intestinal MAIT cells, but not by fetal splenic, intrahepatic and pulmonary MAIT cells ( Fig. 3a ). Taken together, our detailed phenotypic analysis suggests that fetal MAIT cells migrate to and mature in the mucosal tissues and liver. Furthermore, the data support the notion that fetal Vα7.2 + CD161 − T cells are distinct from the developing MAIT-cell population, despite sharing of the TCR Vα7.2 segment. 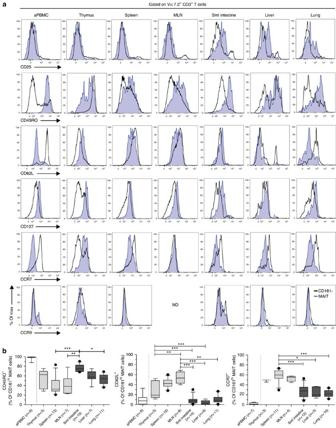Figure 3: Detailed phenotypic analysis of fetal MAIT cells. (a) CD25, CD45RO, CD62L, CD127, CCR7 and CCR9 expression was determined on Vα7.2+CD161hiMAIT cells and Vα7.2+CD161−T cells from fetal tissues and control adult PBMCs from at least three independent donors. Representative FACS plots are shown. (b) Expression of CD45RO, CD62L and CCR7 on MAIT cells is shown in left, middle and right subpanel, respectively. CD45RO expression was determined in the thymus (n=5), spleen (n=13), mesenteric lymph nodes (MLN) (n=7), small (sml) intestine (n=13), liver (n=7) and lung (n=11). CD62L was assessed in the thymus (n=5), spleen (n=12), MLN (n=8), sml intestine (n=14), liver (n=6) and lung (n=11). CCR7 was determined in the thymus (n=3), spleen (n=11), MLN (n=4), sml intestine (n=12), liver (n=5) and lung (n=10). Box and whisker plot shows median, IQR and the 10th to the 90th percentile. *P<0.05, **P<0.01, ***P<0.001 (Kruskal–Wallis ANOVA followed by Dunn’spost-hoctest). Figure 3: Detailed phenotypic analysis of fetal MAIT cells. ( a ) CD25, CD45RO, CD62L, CD127, CCR7 and CCR9 expression was determined on Vα7.2 + CD161 hi MAIT cells and Vα7.2 + CD161 − T cells from fetal tissues and control adult PBMCs from at least three independent donors. Representative FACS plots are shown. ( b ) Expression of CD45RO, CD62L and CCR7 on MAIT cells is shown in left, middle and right subpanel, respectively. CD45RO expression was determined in the thymus ( n =5), spleen ( n =13), mesenteric lymph nodes (MLN) ( n =7), small (sml) intestine ( n =13), liver ( n =7) and lung ( n =11). CD62L was assessed in the thymus ( n =5), spleen ( n =12), MLN ( n =8), sml intestine ( n =14), liver ( n =6) and lung ( n =11). CCR7 was determined in the thymus ( n =3), spleen ( n =11), MLN ( n =4), sml intestine ( n =12), liver ( n =5) and lung ( n =10). Box and whisker plot shows median, IQR and the 10th to the 90th percentile. * P <0.05, ** P <0.01, *** P <0.001 (Kruskal–Wallis ANOVA followed by Dunn’s post-hoc test). Full size image Fetal MAIT cells cycle in vivo and proliferate in vitro Several studies have indirectly suggested that human MAIT cells actively proliferate and expand within the first few years of life [3] , [9] , possibly due to interaction with the commensal microflora established after birth. We therefore investigated expression of the cell proliferation marker Ki67 in fetal MAIT cells ex vivo . Interestingly, MAIT cells from freshly isolated fetal tissues expressed considerable levels of Ki67 ( Fig. 4a ), across fetal tissues examined ( Fig. 4b left). Levels of Ki67 did not correlate with those of CD25 and PLZF. Because fetal CD8αα MAIT cells appear to derive from CD8αβ MAIT cells, we then compared Ki67 levels in both cell populations in fetal small intestine and lung tissues, which had sufficient CD8αα MAIT cells available for this analysis ( Fig. 2c,d ). The CD8αα MAIT-cell population displayed a trend towards fewer Ki67-expressing cells when compared with the CD8αβ MAIT-cell population ( Fig. 4b right). These data together indicate that fetal MAIT cells are cycling in vivo , and that this capacity may be reduced when they mature to the CD8αα stage. 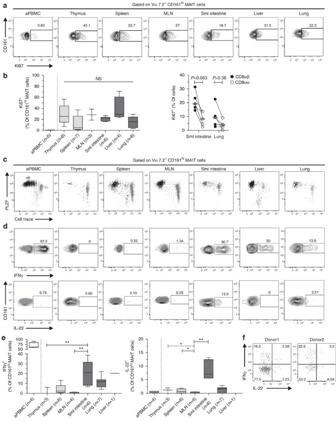Figure 4: Fetal MAIT cells proliferate and produce cytokines following bacterial stimulation. (a,b) Freshly isolated, unstimulated MNCs from fetal tissues and control adult (a) PBMCs were stained intracellularly for Ki67. Inb, left panel, Ki67 is measured in aPBMC (n=5), thymus (n=6), spleen (n=7), mesenteric lymph nodes (MLN) (n=3), small (sml) intestine (n=6), liver (n=4) and lung (n=6). The proportion of Ki67-expressing CD8αα and CD8αβ MAIT cells from fetal small intestine and lung tissues is shown inb, right. Horizontal bars indicate median, and statistical significance was calculated using the Wilcoxon-signed rank test. (c,d) MNCs from fetal tissues and adult PBMCs were stained with Cell Trace, and then cultured with PFA-fixedE. coli+anti-CD28 for 6 days in the presence of IL-2. Alternatively, they were directly stimulated with PFA-fixedE. coli+anti-CD28 overnight, and cytokine production and PLZF expression was assessed by intracellular staining. (e) The proportion of IFNγ and IL-22-expressing MAIT cells in aPBMC (n=4), thymus (n=3), spleen (n=6), MLN (n=4), sml intestine (n=6), lung (n=6) and liver (n=1). (f) IFNγ and IL-22 co-expression from two representative donors. Representative FACS plots are shown. Box and whisker plot shows median, IQR and the 10th to the 90th percentile. *P<0.05, **P<0.01 (Kruskal–Wallis ANOVA followed by Dunn’spost hoctest). Figure 4: Fetal MAIT cells proliferate and produce cytokines following bacterial stimulation. ( a , b ) Freshly isolated, unstimulated MNCs from fetal tissues and control adult (a) PBMCs were stained intracellularly for Ki67. In b , left panel, Ki67 is measured in aPBMC ( n =5), thymus ( n =6), spleen ( n =7), mesenteric lymph nodes (MLN) ( n =3), small (sml) intestine ( n =6), liver ( n =4) and lung ( n =6). The proportion of Ki67-expressing CD8αα and CD8αβ MAIT cells from fetal small intestine and lung tissues is shown in b , right. Horizontal bars indicate median, and statistical significance was calculated using the Wilcoxon-signed rank test. ( c , d ) MNCs from fetal tissues and adult PBMCs were stained with Cell Trace, and then cultured with PFA-fixed E. coli +anti-CD28 for 6 days in the presence of IL-2. Alternatively, they were directly stimulated with PFA-fixed E. coli +anti-CD28 overnight, and cytokine production and PLZF expression was assessed by intracellular staining. ( e ) The proportion of IFNγ and IL-22-expressing MAIT cells in aPBMC ( n =4), thymus ( n =3), spleen ( n =6), MLN ( n =4), sml intestine ( n =6), lung ( n =6) and liver ( n =1). ( f ) IFNγ and IL-22 co-expression from two representative donors. Representative FACS plots are shown. Box and whisker plot shows median, IQR and the 10th to the 90th percentile. * P <0.05, ** P <0.01 (Kruskal–Wallis ANOVA followed by Dunn’s post hoc test). Full size image We next investigated the ability of fetal MAIT cells to proliferate in vitro in response to fixed E. coli stimulation for 6 days. Fetal MAIT cells from all tissues examined proliferated vigorously in response to E. coli stimulation ( Fig. 4c and Supplementary Fig. 2a ). Culture with anti-CD28 and IL-2 alone did not induce significant MAIT-cell proliferation in adult PBMC or full-term fetal cord blood mononuclear cells (CBMC) ( Supplementary Fig. 2b ). In addition, the MAIT-cell proliferation induced by both fixed whole-cell E. coli and E. coli supernatants was MR1 dependent ( Supplementary Fig. 2b ). MAIT cells from fetal tissues and adult blood were also able to proliferate in response to PHA stimulation, although at a considerably lower magnitude ( Supplementary Fig. 2c ). Interestingly, MAIT-cell proliferation was associated with high PLZF levels in both E. coli -stimulated and PHA-stimulated cultures ( Fig. 4c and Supplementary Fig. 2c ), consistent with the notion that PLZF drives MAIT-cell maturation and function. Furthermore, fetal CD8α + Vα7.2 + CD161 hi MAIT cells that had proliferated extensively in vitro (Cell Trace lo ) were primarily CD8αβ ( Supplementary Fig. 2d ), further strengthening the notion that the proliferative capacity of fetal CD8αα MAIT cells is inferior to that of fetal CD8αβ MAIT cells. Taken together, these data suggest that fetal MAIT cells are cycling in vivo and are highly proliferative in response to bacterial antigen stimulation. Acquisition of IFNγ and IL-22 during maturation and homing Finally, we examined the fetal MAIT-cell response to an overnight exposure to E. coli in vitro . Adult peripheral blood MAIT cells produced high levels of IFNγ, as previously described [3] , [8] , [11] , [15] , [24] . In contrast, MAIT cells from the fetal thymus, spleen and MLN were unable to produce appreciable levels of IFNγ following stimulation with E. coli ( Fig. 4d,e left). This was probably not due to an intrinsic deficiency per se , as PMA/ionomycin stimulation was able to elicit IFNγ production ( Supplementary Fig. 2e left) but maybe rather due to their immature differentiation stage. MAIT cells from the fetal small intestine, liver and lung produced moderate levels of IFNγ following E. coli stimulation ( Fig. 4d,f ). Most notably, fetal intestinal MAIT cells and, to a much lesser extent, fetal pulmonary MAIT cells were able to produce the tissue protective cytokine IL-22 following E. coli stimulation ( Fig. 4d,e right,f). This pattern held true after PMA/ionomycin stimulation of cells from the same donors ( Supplementary Fig. 2e right), suggesting that IL-22 production is restricted to intestinal fetal MAIT cells. Of note, a significant proportion of IL-22 + intestinal MAIT cells also produced IFNγ ( Fig. 4f ). Because of the restricted numbers of fetal MAIT cells, and limited biological material, we were unable to investigate possible differences in cytokine expression patterns between MAIT-cell subsets. However, in a few donors where MAIT-cell numbers were sufficient to perform such analysis, there was no significant difference in cytokine production between CD8 + and DN MAIT-cell subsets. Taken together, these results indicate that fetal MAIT cells from the small intestine, liver and lung develop responsiveness against bacteria before establishment of commensal microflora and before overt bacterial exposure. This innate-like responsiveness is consistent with the pattern of MAIT-cell maturation in these organs ( Fig. 5 ). 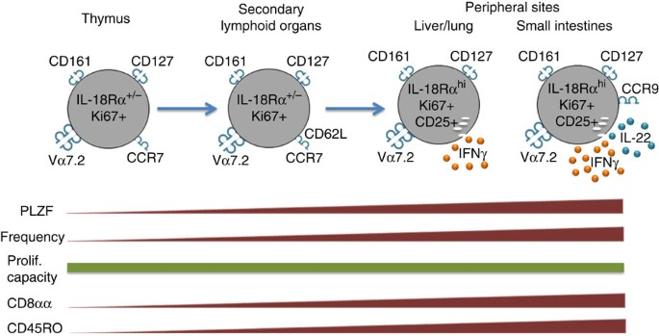Figure 5: Gradual maturation of human fetal MAIT cells in lymphoid and peripheral organs. Summary illustration of phenotypic and functional changes in MAIT cells developing and maturing in tissues of the human fetus. Figure 5: Gradual maturation of human fetal MAIT cells in lymphoid and peripheral organs. Summary illustration of phenotypic and functional changes in MAIT cells developing and maturing in tissues of the human fetus. Full size image The MR1-restricted MAIT cells are a relatively recently described, and highly evolutionarily conserved, invariant T-cell subset with innate-like capacity to rapidly respond to a range of microbes. Studies of MAIT cells in human fetal development are important for the understanding of their fundamental immunobiological characteristics, as well as for the role these cells play in the fetus and the newborn. Here, we have investigated the development and maturation of MAIT cells in second trimester human fetal tissues. Vα7.2 + CD161 hi MAIT cells are present in both CD3 lo and CD3 hi thymocytes at 18 weeks post gestation as an almost exclusively CD8αβ population with low levels of PLZF and IL-18Rα. MAIT cells in secondary lymphoid organs, such as the spleen and MLN, express PLZF but do not universally co-express IL-18Rα. In contrast, in the fetal small intestine, liver and lung, MAIT cells are present at a higher frequency and display a mature phenotype including IL-18Rα, high levels of PLZF, and CD8αα. MAIT cells in all organs express Ki67 in vivo and readily proliferate in response to E. coli in vitro . Finally, intestinal, lung and liver fetal MAIT cells have gained the capacity to produce IFNγ following recognition of E. coli , with IL-22 production apparently restricted to the small intestines. Together, these data define the gradual post-thymic maturation pathway, and the acquisition of innate-like antimicrobial responsiveness, in MAIT cells developing in the second trimester human fetus ( Fig. 5 ). The relatively high levels of Ki67 expression and proliferative responses in fetal MAIT cells are in sharp contrast to the phenotype exhibited by MAIT cells in adult peripheral blood. This fetal MAIT cell proliferation is paired with consistently high expression of CD127 and may at least partly represent homeostatic expansion of MAIT cells to fill their niche in the developing immune system. In spleen and MLN, this highly proliferative state is associated with a relatively immature phenotype with low CD25 expression and modest levels of CD45RO and IL-18Rα. Similarly, levels of the transcription factor PLZF, associated with effector function in innate-like T cells in mice [28] , remain low in the spleen and MLN. Accordingly, MAIT cells in these organs produce very little IFNγ following stimulation with E. coli . All these observations are consistent with an immature and highly proliferative developmental stage in splenic and lymph node MAIT cells in the fetus. This picture is vastly different in the peripheral sites we have investigated, the small intestines, liver and lung. At these sites, the Vα7.2 + CD161 hi MAIT cells have gained high expression of PLZF and acquired expression of IL-18Rα. MAIT cells in these sites also comprise a significant CD8αα-expressing population, are CD45RO + and express CD25. At the same time, they maintain a degree of Ki67 expression and the ability to proliferate in response to E. coli , albeit at what appears to be a lower level than in lymphoid organs. This mature phenotype is most distinct in the small intestine, and this is also where IFNγ production in response to E. coli is the highest. The second trimester small intestine, and also the lung and liver, thus have a MAIT-cell population that exhibit a phenotype consistent with mature MAIT cells in the adult human, with the important difference that their proliferative capacity is higher. It should be noted, however, that MAIT cells from adult peripheral blood also have some ability to proliferate in response to E. coli plus IL-2 stimulation. This is in contrast to several published studies that suggested MAIT cells from adult peripheral blood have poor proliferative capacity [3] , [10] , [24] , [25] . One difference between the present study and these previous studies is that we utilized whole-cell bacterial stimulation in combination with exogenous IL-2, instead of anti-CD3/CD28 or PHA stimulations in the absence of IL-2. A recent study suggests that pro-inflammatory cytokines produced by APC in response to bacterial stimulation including IL-18 and IL-12 can activate MAIT cells independent of TCR ligation [29] . Thus, it is also possible that IL-18 and IL-12 contribute to MAIT cell proliferation in vitro , as previously reported [24] , [25] . Small intestinal fetal MAIT cells respond to E. coli by production of not only IFNγ but also of IL-22. Expression of this cytokine was not observed in other tissues, with the exception of minute levels detected in the lung, and this suggests that MAIT cells in the small intestines are programmed by their environment to exhibit a more diverse functional profile. In murine models, retinoic acid, IL-1β and IL-23 are produced by intestinal mucosa resident DCs particularly during bacterial infection and inflammation [30] , [31] , [32] , [33] and can enhance IL-22 production by murine intestinal innate lymphocyte populations, including γδT cells and innate lymphoid cells (ILCs) [31] , [34] . It is tempting to speculate that such factors can also be produced by human fetal intestinal resident DCs and enhance IL-22 production by MAIT cells following E. coli stimulation in vitro . IL-22R1 is expressed by epithelial cells and keratinocytes among other cells, and IL-22 induces expression of antimicrobial peptides in these cells [35] (reviewed in ref. 36 ). IL-22 −/− mice display increased intestinal epithelial damage and susceptibility to certain bacterial infections [37] . The observation that MAIT cells express IL-22 points to that these cells may play a role in maintaining intestinal mucosal tissue defence and integrity. Furthermore, this function develops already at the fetal second trimester stage. Murine models have suggested that the post-natal commensal microflora is necessary for MAIT-cell maturation. The present data clearly indicate that this is not the case for humans. What factors drive MAIT-cell maturation in the human fetus is unclear, but it is tempting to speculate in three directions. One possibility is that an endogenous stimulatory MR1-presented ligand is present and available at the mucosal sites. For example, a partial TCR agonist might provide sufficient stimuli for MAIT-cell selection, survival and maturation. Such a ligand could, in the cytokine milieu and conditions that exist within the fetal microenvironment, provide a strong enough stimulus for maturation of the developing MAIT-cell population. Another possibility is that the fetal mucosa is exposed to components of the microbial riboflavin biosynthetic pathway that are of maternal origin and ultimately derived from the mother’s commensal microflora. The amniotic fluid could, at least theoretically, be a carrier of such stimulatory MAIT cell ligands. A third aspect that may influence the maturation at peripheral sites is that developing MAIT cells going into these sites may be under less influence by FoxP3 + T-regulatory (Treg) cells. It was previously shown that fetal lymphoid organs are rich in Treg cells [38] , [39] . In any case, the association between maturation and gain of functions, and upregulation of PLZF expression argues for the involvement of an MR1-presented ligand, as it has previously been shown that PLZF expression is induced by TCR engagement [40] . Pre-natal development of mature MAIT cells and their enrichment and location at the mucosal barriers in the intestines and lung may be important for immune protection of the fetus, and perhaps even more so, of the newborn child. The newborn is immediately exposed to a plethora of microbes, including bacteria, fungi and viruses. Whereas maternal antibodies transferred via the placenta and breast milk are critical, they will probably not offer protection against all kinds of pathogens. Cellular immune mechanisms with innate characteristics that are ready to recognize microbes at mucosal surfaces at the time of birth may be very important, and this provides a possible evolutionary rationale behind the presence of mature MAIT cells in the fetal small intestine and lung. MAIT cells can thus contribute to the innate protection of the host together with cells such as the ILCs and the invariant natural killer T (iNKT) cells that develop early during ontogeny [41] , [42] . Interestingly, MAIT cells were recently found to be critical for optimal mucosal immune responses during in vivo pulmonary bacterial infection in a mouse model [19] . The present study delineates the development of human MAIT cells before birth and establishment of mucosal microbiota. The findings define the gradual maturation pathway of MAIT cells in lymphoid and peripheral organs and the acquisition of innate-like antimicrobial activity of MAIT cells in human fetal intestinal mucosa before birth. Given the broad spectrum of microbes recognized by MAIT cells, the establishment and maturation of this arm of immunity before birth may help protect the mucosal surfaces of the newborn from a range of pathogenic microbes. Human subject and tissues Healthy, HIV-uninfected adults were recruited at the Division of Experimental Medicine, San Francisco General Hospital (SFGH). Human fetal tissues (the thymus, spleen, MLN, small intestine, liver and lung) were collected from second trimester elective abortions from The SFGH Women’s Options Center (San Francisco, CA). Several fetal thymi were from Advanced Bioscience Resources (Alameda, CA). Fetal tissues were collected from gestational weeks 18–23. Written informed consent was obtained from all individuals in accordance with study protocols conforming to the provisions of the Declaration of Helsinki and approved by the Institutional Review Board, the Committee on Human Subjects Research, UCSF, and the Regional Ethics Review Board in Stockholm. Peripheral blood and fetal tissue processing Fetal organs were collected into cold RPMI medium with 10% FCS, 25 mM HEPES, penicillin, streptomycin and L -glutamine (RF10 medium), and kept on ice. Fetal (15–30) MLNs were collected from the mesentery with fine-pincer forceps. Fetal small intestines were cut into 6-cm long sections, and the meconium was removed by making a longitudinal incision along the tissue section and gently scrapping away the material with a cell scrapper, followed by incubation in RF10 medium at 37 °C for 10 min with frequent, gentle agitations to remove residual meconium. Fetal liver and lung were cut into small pieces using scalpels. The fetal small intestine, liver, lung and MLN were subsequently incubated for 50 min at 37 °C in serum-free RPMI medium with 0.25 mg ml −1 type II collagenase (Sigma-Aldrich), with 30 s vigorous vortexing every 10 min. Collagenase treatment was terminated by adding cold RF10 medium. Fetal small intestine, liver and lung cell suspensions were filtered through 70 μm cell strainers (BD Biosciences), washed twice with 50 ml of PBS and resuspended in cold RF10 medium. Fetal spleens and thymi were passed through a 70 μm cell strainer and resuspended in cold RF10 medium. Adult PBMC and fetal MNC from the spleen, small intestine, liver, lung and cord blood were isolated by Ficoll-Hypaque density gradient centrifugation (GE Healthcare). Following isolation, cells were washed twice in PBS, counted and immediately used for staining and/or functional assays. Functional assay MAIT cell functions were determined in vitro using a paraformaldehyde-fixed E. coli stimulation (DH5α strain, multiplicity of infection 6) in the presence of 1.25 μg ml −1 anti-CD28 mAb (BD Biosciences) [11] . Cells were cultured overnight at 37 °C/5% CO 2 , and monensin (Golgi Stop, BD Biosciences) was added during the last 6 h of incubation. In selected experiments, cells were stained with 5 μM Cell Trace Violet Cell Proliferation Kit (Invitrogen) as per the manufacturer’s instructions and cultured with fixed E. coli in the presence of anti-CD28 as described, or with 1 μg ml −1 phytohemagglutinin (PHA; Sigma), in RF10 medium supplemented with 50 μg ml −1 gentamicin (Gibco). After 24 h, recombinant human IL-2 (Roche) was added at a final concentration of 50 IU ml −1 and replenished every 48 h. MAIT-cell proliferation was determined by flow cytometry 6 days after E. coli feeding or PHA stimulation. Flow cytometry Anti-CD14 and anti-CD19 APC-H7 (both at 1:100), anti-CD25 PECy7 (1:50), anti-CD62L V450 (1:50), anti-CD127 PECy7 (1:100), anti-CD161 FITC (1:10), anti-IFNγ V450 (1:200), anti-Ki67 FITC (1:10) were from BD Biosciences. Anti-CD3 ECD (1:100) and anti-CD8β PE (1:50) were from Beckman Coulter. Anti-Vα7.2 FITC (1:10) and PE (1:20), anti-CD45 Alexa Fluor 700 (1:400), anti-CD45RO PECy7 (1:50), anti-CCR9 Alexa Fluor 647 (1:20), anti-Ki67 Brilliant Violet 421 (1:20), anti-CCR7 Brilliant Violet 421 (1:20) were from BioLegend. Anti-CD161 PerCP-Cy5.5 (1:20), anti-IL-22 PerCP-eFluor 710 (1:50) were from eBioscience. Anti-IL-18R PE (1:20), and anti-PLZF APC (1:10) were from R&D systems. Anti-CD4 Qdot 655 (1:400), anti-CD8α Qdot 605 (1:800), anti-CD45 Qdot 705 (1:100), live/dead aqua (1:100) and near infrared fixable (1:400) cell stain were from Invitrogen. Cell surface staining was performed using directly conjugated antibodies and fixed in Cytofix/Cytoperm (BD Biosciences). Intracellular staining was performed using the appropriate mAb’s in Perm/Wash (BD Biosciences). Samples were acquired on an LSRII flow cytometer (BD Biosciences) equipped with 405, 488, 532 and 647 nm lasers. Single-stained polystyrene beads (BD Biosciences) were used for compensation purposes. Software-based compensation was performed using the compensation platform in FlowJo software version 9.5 (Tree Star). Statistical analyses Continuous variables were first assessed for normality, and differences in independent samples were assessed using t -test or Mann–Whitney test for continuous variables as appropriate. The Kruskal–Wallis analysis of variance (ANOVA) followed by Dunn’s post hoc test, or one-way ANOVA followed by Bonferroni’s post hoc test was used to detect differences across multiple samples. The Wilcoxon-signed rank test was used to determine significance between paired samples. Correlations were evaluated using Spearman’s rank correlation. Statistical analyses were performed using Prism version 5 (GraphPad), and two-sided P -values<0.05 were considered significant. Control adult PBMCs were included for comparison purposes only and excluded from all statistical analyses. How to cite this article: Leeansyah, E. et al. Acquisition of innate-like microbial reactivity in mucosal tissues during human fetal MAIT-cell development. Nat. Commun. 5:3143 doi: 10.1038/ncomms4143 (2014).